Imaging regulatory T cell dynamics and CTLA4-mediated suppression of T cell priming Foxp3 + regulatory T cells (Tregs) maintain immune homoeostasis through mechanisms that remain incompletely defined. Here by two-photon (2P) imaging, we examine the cellular dynamics of endogenous Tregs. Tregs are identified as two non-overlapping populations in the T-zone and follicular regions of the lymph node (LN). In the T-zone, Tregs migrate more rapidly than conventional T cells (Tconv), extend longer processes and interact with resident dendritic cells (DC) and Tconv. Tregs intercept immigrant DCs and interact with antigen-induced DC:Tconv clusters, while continuing to form contacts with activated Tconv. During antigen-specific responses, blocking CTLA4-B7 interactions reduces Treg–Tconv interaction times, increases the volume of DC:Tconv clusters and enhances subsequent Tconv proliferation in vivo . Our results demonstrate a role for altered cellular choreography of Tregs through CTLA4-based interactions to limit T-cell priming. Regulatory T cells (Tregs) expressing the Foxp3 transcription factor constitute a critical component of peripheral immune homoeostasis and tolerance. Several autoimmune and inflammatory pathologies in humans are associated with functional defects in Tregs, and depletion of Tregs in experimental animals leads to systemic autoimmune and allergic disease accompanied by unchecked lymphoproliferation [1] , [2] , [3] , [4] . Expression of an inhibitory member of the immunoglobulin super-family cytotoxic T-lymphocyte antigen 4 (CTLA4) by Tregs is critical for their function. The loss of Treg-specific CTLA4 expression or treatment with a blocking antibody lead to potentially lethal T-cell-mediated autoimmune pathology [5] , [6] , [7] , [8] . Moreover, polymorphisms in human CTLA4 are linked to the development of autoimmune diseases, including type I diabetes and primary progressive multiple sclerosis [9] . Although it is now established that Tregs and their expression of CTLA4 are both indispensable for the maintenance of immune homoeostasis [4] , [5] , [6] , [10] , the underlying cellular and molecular mechanisms of CTLA4-mediated suppression are not well-understood [11] . In vitro studies of T-cell cultures in the absence of antigen-presenting cells (APC) have demonstrated that Tregs directly suppress both CD4 + and CD8 + T-cell proliferation in a contact-dependent, antigen-independent manner [12] , [13] . However, in vivo data are lacking on how endogenous Tregs interact with APCs and conventional T cells (Tconvs). Two-photon (2P) microscopy allows detailed observation and analysis of the spatio-temporal choreography of live cell–cell interactions within the native tissue environment of the lymph node (LN), secondary lymphoid organs and peripheral tissues [14] , [15] . In the LN, naive CD4 + T cells exhibit three distinct phases of behaviour in relation to dendritic cells (DCs) during initiation of an immune response [16] : (1) dynamic scanning with transient interactions with antigen-bearing DCs; (2) formation of dynamic clusters in which multiple T cells stop migrating freely and form stable contacts with DCs and (3) disengagement of T cells from DCs, followed by swarming behaviour and subsequent antigen-specific T-cell proliferation. Previous 2P imaging studies have investigated Treg-induced suppression during T-cell priming either by addition of in vitro -separated CD4 + CD25 + T cells [17] , [18] , [19] , [20] , [21] or by diphtheria toxin-induced depletion of Tregs [22] . Notably, no previous studies have imaged endogenous Tregs in the context of both Tconvs and DCs. Simultaneous and direct imaging of endogenous Tregs together with naïve T cells and DCs would permit insight into the cellular behaviour and in vivo mechanisms that underlie immunoregulation. Here using 2P microscopy of LNs from Foxp3 EGFP mice, we have characterized the dynamics of unperturbed, endogenous Tregs interacting with Tconv and with DCs under steady-state conditions, in the presence of LPS-activated DCs as a model for inflammation and during antigen-specific CD4 T-cell priming. We further demonstrate the crucial involvement of CTLA4-B7 interactions in determining cellular dynamics among Tregs, Tconvs and DCs in vivo . Imaging regional differences in Treg dynamics To visualize endogenous Treg cells, we screened mouse strains that express fluorescent proteins specific to Tregs, and identified Foxp3 EGFP mice as optimal for 2P imaging. Developed by Haribhai et al . [23] , Foxp3 EGFP mice contain a bicistronic Foxp3–enhanced green fluorescent protein (Foxp3–EGFP) gene that induces reliable co-expression of EGFP and Foxp3 in bona fide endogenous Tregs. EGFP + Tregs were clearly visualized by 2P imaging of explanted LNs without exogenous labelling or adoptive transfer ( Fig. 1a ). Mapping the distribution of Tregs with respect to CFP + CD19 + B cells and CMTMR-labelled CD4 + CD25 − T (Tconv) cells revealed that Tregs are abundant in the T-cell zone, and are also present at lower density within B-cell follicles and in the sub-capsular space ( Fig. 1b , Supplementary Video 1 ). Time-lapse images of Tregs and associated tracks indicated little or no active exchange between follicle and adjacent T-zone ( Fig. 1c and Supplementary Video 2 ). Their basal motility characteristics, morphology and choreography clearly differed between locations within the LN. Mean velocities of Tregs in the T-cell zone (14.6±0.2 μm min −1 ) were significantly higher than follicular Tregs (fTregs; 12.9±0.1 μm min −1 , P <0.001). Near or at the capsule, Tregs migrated more slowly (9.5±0.2 μm min −1 ; Fig. 1d ), many along collagen fibres ( Supplementary Fig. 1a and Supplementary Video 3 ). The collagen-interacting Tregs migrated more slowly than other Tregs within 50 μm of the capsule ( Supplementary Fig. 1b ). Deeper in the paracortex (>50 μm below the capsule), Tregs moved rapidly and extended the cellular processes ( Fig. 1e and Supplementary Video 4 ). Within the T-cell zone, Tregs exhibited higher mean velocities (13.9±0.2 μm min −1 ) than colocalized Tconv cells (12.0±0.2 μm min −1 , P <0.001; Fig. 1f ). Moreover, Tregs extended longer cellular processes than colocalized Tconvs ( Supplementary Fig. 1c ); and fTregs were, on average, even more elongated ( Supplementary Fig. 1d ). Close examination under steady-state conditions in the absence of antigen revealed cell–cell contacts between Treg and Tconv cells ( Fig. 1g ). 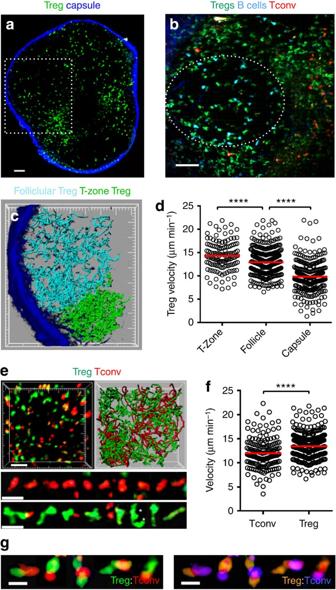Figure 1: Endogenous Foxp3+Treg regional behaviour and interaction with Tconvs. (a) Tregs in inguinal lymph node from a Foxp3EGFPmouse under steady-state conditions. Green, EGFP+endogenous Tregs; blue, second-harmonic collagen signal in capsular boundary. Single plane image, scale bar, 100 μm. White square represents area imaged inc. SeeSupplementary Video 2. (b) T-zone and follicular Tregs (both green), visualized 72 h after adoptive transfer of CFP+CD19+B cells (blue) and CMTMR-labelled Tconv cells (red). Note: Tregs colocalized with B cells within the dotted outline and at higher density with Tconv cells throughout the T-cell zone. Scale bar, 50 μm. (c) Non-overlapping populations of Tregs in the T-zone and the follicle. Treg movements represented by tracks within (light blue tracks) and outside the B-cell follicle (bright green). Cells tracked over 29:38 (min:s); 35-μmz-stack 50-μm tick marks. (d) Treg velocities in three regions of the lymph node. Each circle represents mean velocity in the T-cell zone (n=174 tracks), in the follicle (n=397 tracks), and within 50 μm of the capsule (n=343 tracks). Data pooled from four experiments. Open circles represent measurements from individual cell tracks; red bars indicate overall mean values andPvalues are marked in the figures as *P<0.05, **P<0.01, ***P<0.001 and ****P<0.0001 using Mann–WhitneyU-test. (e) CMTMR-labelled Tconv cells adoptively transferred 24 h before imaging and tracked with Tregs over 12 min. Still image (top left, scale bar, 30 μm) and corresponding tracks (top right) of Tconv cells (red) and Tregs (green) in the T-zone. Lower panels: magnified views of representative individual Tconv cells and endogenous Tregs (scale bar, 20 μm). Asterisks mark cellular processes. SeeSupplementary Video 4. (f) Velocities of individual Tregs (n=217 tracks) and Tconvs (n=166 tracks) in the T-zone. Data pooled from three experiments. (g) Tconvs (red) and Tregs (green) in the absence of antigen; right panel pseudocoloured to highlight areas of contact; scale bar, 10 μm. Figure 1: Endogenous Foxp3 + Treg regional behaviour and interaction with Tconvs. ( a ) Tregs in inguinal lymph node from a Foxp3 EGFP mouse under steady-state conditions. Green, EGFP + endogenous Tregs; blue, second-harmonic collagen signal in capsular boundary. Single plane image, scale bar, 100 μm. White square represents area imaged in c . See Supplementary Video 2 . ( b ) T-zone and follicular Tregs (both green), visualized 72 h after adoptive transfer of CFP + CD19 + B cells (blue) and CMTMR-labelled Tconv cells (red). Note: Tregs colocalized with B cells within the dotted outline and at higher density with Tconv cells throughout the T-cell zone. Scale bar, 50 μm. ( c ) Non-overlapping populations of Tregs in the T-zone and the follicle. Treg movements represented by tracks within (light blue tracks) and outside the B-cell follicle (bright green). Cells tracked over 29:38 (min:s); 35-μm z -stack 50-μm tick marks. ( d ) Treg velocities in three regions of the lymph node. Each circle represents mean velocity in the T-cell zone ( n =174 tracks), in the follicle ( n =397 tracks), and within 50 μm of the capsule ( n =343 tracks). Data pooled from four experiments. Open circles represent measurements from individual cell tracks; red bars indicate overall mean values and P values are marked in the figures as * P <0.05, ** P <0.01, *** P <0.001 and **** P <0.0001 using Mann–Whitney U -test. ( e ) CMTMR-labelled Tconv cells adoptively transferred 24 h before imaging and tracked with Tregs over 12 min. Still image (top left, scale bar, 30 μm) and corresponding tracks (top right) of Tconv cells (red) and Tregs (green) in the T-zone. Lower panels: magnified views of representative individual Tconv cells and endogenous Tregs (scale bar, 20 μm). Asterisks mark cellular processes. See Supplementary Video 4 . ( f ) Velocities of individual Tregs ( n =217 tracks) and Tconvs ( n =166 tracks) in the T-zone. Data pooled from three experiments. ( g ) Tconvs (red) and Tregs (green) in the absence of antigen; right panel pseudocoloured to highlight areas of contact; scale bar, 10 μm. Full size image In summary, under steady-state conditions two non-overlapping populations of Tregs explore the T-zone and the follicle. fTregs have been identified previously as CD4 + Foxp3 + cells expressing CXCR5 and Bcl6 (refs 24 , 25 ). Endogenous Tregs in the T-cell zone are the most rapidly motile cells in the LN reported to date. In the remainder of this report, we focus on the dynamics of Tregs interacting with Tconvs and DCs in the T-zone. Tregs engage resident DCs and Tconv cells To image endogenous Tregs, resident DCs and Tconvs simultaneously, we crossed Foxp3–eGFP male mice with CD11c–enhanced yellow fluorescent protein (CD11c–EYFP) reporter female mice [26] . In the resultant F1 heterozygote females, 50% of Foxp3 + Tregs express EGFP [23] , and EYFP is highly expressed in the LN-resident DCs. CMTMR-labelled Tconv cells were then adoptively transferred into these F1 mice, followed by LN imaging 24 h after cells were allowed to equilibrate ( Fig. 2a ). The highly dynamic endogenous Tregs ( Fig. 2b,c and Supplementary Video 5 ) interacted with CD11c–EYFP + resident DCs, forming transient contacts that lasted longer (3.3±0.4 min) than interactions between Tconvs and DCs (2.5±0.3 min, P <0.004, Fig. 2d ). In the female heterozygous recipient population, only half of the Tregs are GFP + ; therefore, the actual mean frequency of Treg:DC contacts would be twice that observed ( Fig. 2e ). Thus, a single DC makes contact with 8.6±1.1 Tregs per hour. Given the mean frequency of contacts between endogenous Tregs and resident DCs and their average contact duration of 3.3 min, our measurements indicate that a LN-resident DC is in contact with at least one Treg for 28.4 min per hour—that is, nearly half of the time. Conventional CD4 T cells briefly interacted with Tregs under basal conditions, encountering up to 13.4 Tregs per hour ( Fig. 2e ) for an average of 1:36 (min:s). Therefore, a single Tconv cell spends an average of 21.5 min per hour (36% of the time) in contact with endogenous Tregs. These results demonstrate that individual Tregs, although less abundant than Tconv cells, are highly active and frequently encounter both DCs and Tconv under basal conditions. 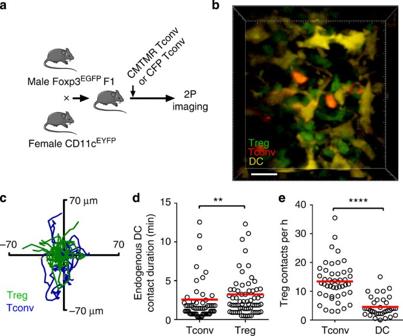Figure 2: Tregs interact with LN-resident DCs. (a) Experimental design to visualize endogenous Tregs together with resident DCs and Tconv cells. CMTMR-labelled Tconv cells from WT C57Bl/6 mice or CFP+Tconv cells from β-actin–CFP mice were adoptively transferred 12 h or 4 days, respectively, prior to imaging, into F1 of Foxp3EGFP× CD11cEYFPmice. (b) Interactions among Tconv cells (red), resident DCs (yellow) and Tregs (green) under steady-state conditions. Scale bar, 20 μm, seeSupplementary Video 5. (c) Superimposed Treg (green) and Tconv (blue) tracks,zcompressed and normalized to DC position at the centre (x,y=0, 0). Data from CFP+Tconv cells are shown; similar results were obtained with CMTMR-labelled Tconv cells. Cells were tracked over 15:21 (min:s). (d) Contact durations between cell pairs: Tconvs interacting with DCs (n=61); Tregs interacting with DCs (n=67). Data from CFP+Tconv cells are shown, and are also representative of results with CMTMR-labelled Tconv cells. Three independent experiments, imaging duration >1 h. (e) Observed contact frequencies with endogenous Tregs by labelled Tconvs (n=47) and by resident DCs (n=36), two experiments. Figure 2: Tregs interact with LN-resident DCs. ( a ) Experimental design to visualize endogenous Tregs together with resident DCs and Tconv cells. CMTMR-labelled Tconv cells from WT C57Bl/6 mice or CFP + Tconv cells from β-actin–CFP mice were adoptively transferred 12 h or 4 days, respectively, prior to imaging, into F1 of Foxp3 EGFP × CD11c EYFP mice. ( b ) Interactions among Tconv cells (red), resident DCs (yellow) and Tregs (green) under steady-state conditions. Scale bar, 20 μm, see Supplementary Video 5 . ( c ) Superimposed Treg (green) and Tconv (blue) tracks, z compressed and normalized to DC position at the centre ( x , y =0, 0). Data from CFP + Tconv cells are shown; similar results were obtained with CMTMR-labelled Tconv cells. Cells were tracked over 15:21 (min:s). ( d ) Contact durations between cell pairs: Tconvs interacting with DCs ( n =61); Tregs interacting with DCs ( n =67). Data from CFP + Tconv cells are shown, and are also representative of results with CMTMR-labelled Tconv cells. Three independent experiments, imaging duration >1 h. ( e ) Observed contact frequencies with endogenous Tregs by labelled Tconvs ( n =47) and by resident DCs ( n =36), two experiments. Full size image Activated migratory DCs are intercepted by Tregs Resident DCs in the LN constitutively present low levels of self-antigens, and the T-cell receptor (TCR) repertoire of Tregs is skewed towards self-antigen recognition [27] , [28] . Accordingly, we sought to define the interactions between Tregs and activated, migratory DCs from the periphery. Subcutaneous injection of CMTMR-labelled lipopolysaccharide (LPS)-activated bone marrow-derived DCs (LPS-DCs) into a Foxp3–EGFP animal followed by imaging at 24 h revealed the highest density of DCs on and around collagen fibres just under the LN capsule ( Fig. 3a ). In this region of the LN, Tregs readily interacted with and surrounded immigrant DCs, while forming both brief and extended LPS-DC:Treg contacts ( Fig. 3b ). Strikingly, some Tregs established long-lived (up to 40 min) contacts with LPS-DCs near the capsule ( Fig. 3c,d and Supplementary Video 6 ). 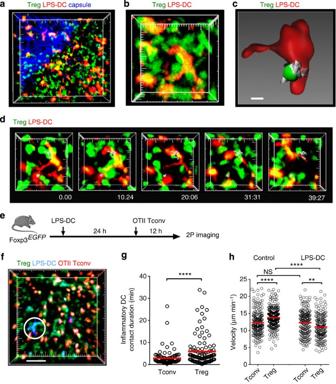Figure 3: Tregs engage immigrant DCs near the lymph node capsule. (a) LPS-activated CMTMR-labelled DCs (red) imaged in the draining inguinal lymph node 24 h after subcutaneous injection into a Foxp3EGFPmouse, showing immigrant DCs encountering and making contact with numerous endogenous Tregs (green) directly beneath the collagen capsule (blue) of the lymph node (major tick marks=20 μm, 50 μmz-stack). SeeSupplementary Video 6. (b) Close-up image of a DC (red) near the collagen capsule and its interactions with several Tregs (green). Major tick marks=10 μm. (c) Space-filled rendering of the DC (red) fromband an associated Treg (green) with track (grey, 39:27 (min:s) duration of imaging), showing close association between Treg and DC (scale bar, 5 μm). (d) Time sequence (times shown in min:s) showing interactions of Tregs (green with grey tracks) engaging recently immigrated DCs (red). (e) Experimental design to examine the effect of LPS-activated DCs on OTII Tconv cells and Tregs. LPS-activated DCs from an ECFP mouse were injected into a Foxp3EGFPmouse followed by adoptive transfer of CMTMR-labelled OTII Tconv cells at 24 h and 2P imaging in the draining lymph node 12 h later. (f) Snapshot showing adoptively transferred OTII Tconv cells (red), LPS-activated DC (blue) and Tregs (green). Scale bar, 30 μm. SeeSupplementary Video 7. (g) Contact durations of Tregs with LPS-DCs (n=110 contacts) and Tconvs with LPS-DCs (88 contacts). Data pooled from three experiments each. (h) Effect of LPS-activated DCs on Treg velocities. Control velocities in the absence of LPS-DCs: Tregn=296; OTII Tconv cellsn=213. In the presence of LPS-DCs, OTII Tconv-cell velocity did not change appreciably (P=0.7,n=207, Mann–WhitneyU-test), whereas Treg velocity was reduced (n=193). Data pooled from three experiments each. NS, not significant. Figure 3: Tregs engage immigrant DCs near the lymph node capsule. ( a ) LPS-activated CMTMR-labelled DCs (red) imaged in the draining inguinal lymph node 24 h after subcutaneous injection into a Foxp3 EGFP mouse, showing immigrant DCs encountering and making contact with numerous endogenous Tregs (green) directly beneath the collagen capsule (blue) of the lymph node (major tick marks=20 μm, 50 μm z -stack). See Supplementary Video 6 . ( b ) Close-up image of a DC (red) near the collagen capsule and its interactions with several Tregs (green). Major tick marks=10 μm. ( c ) Space-filled rendering of the DC (red) from b and an associated Treg (green) with track (grey, 39:27 (min:s) duration of imaging), showing close association between Treg and DC (scale bar, 5 μm). ( d ) Time sequence (times shown in min:s) showing interactions of Tregs (green with grey tracks) engaging recently immigrated DCs (red). ( e ) Experimental design to examine the effect of LPS-activated DCs on OTII Tconv cells and Tregs. LPS-activated DCs from an ECFP mouse were injected into a Foxp3 EGFP mouse followed by adoptive transfer of CMTMR-labelled OTII Tconv cells at 24 h and 2P imaging in the draining lymph node 12 h later. ( f ) Snapshot showing adoptively transferred OTII Tconv cells (red), LPS-activated DC (blue) and Tregs (green). Scale bar, 30 μm. See Supplementary Video 7 . ( g ) Contact durations of Tregs with LPS-DCs ( n =110 contacts) and Tconvs with LPS-DCs (88 contacts). Data pooled from three experiments each. ( h ) Effect of LPS-activated DCs on Treg velocities. Control velocities in the absence of LPS-DCs: Treg n =296; OTII Tconv cells n =213. In the presence of LPS-DCs, OTII Tconv-cell velocity did not change appreciably ( P =0.7, n =207, Mann–Whitney U -test), whereas Treg velocity was reduced ( n =193). Data pooled from three experiments each. NS, not significant. Full size image To investigate LPS-DCs and Tregs in the presence of antigen-specific T cells but in the absence of cognate antigen, we transferred labelled OTII cells ( Fig. 3e ) and observed that LPS-DCs were surrounded by endogenous Tregs ( Fig. 3f and Supplementary Video 7 ). Under these conditions, average Treg contact durations with LPS-DCs were significantly longer ( Fig. 3g ; 5:53±0:38 (min:s)), as compared with both Tconv:LPS-DC (2:53±0:22 (min:s)) and basal Treg:DC interactions (3:14±0:28, both P <0.001; see for example, Figs 2d and 3g ). Consistent with results from wild-type (WT) Tconv cells, endogenous Treg velocities were significantly higher than adoptively transferred OTII Tconv cells; however, endogenous Tregs slowed significantly as they interacted with LPS-DCs, while OTII T-cell velocities were unaltered ( Fig. 3h ). These results led us to examine whether the Treg:DC interactions visualized near the LN capsule may lead to the activation of endogenous Tregs [29] , [30] . Indeed, a higher percentage of CD4 T cells were CD69 + Foxp3 + in animals injected with LPS-DCs, compared with control animals ( Supplementary Fig. 2 ). Contralateral LNs also had an increased number of CD69 + Foxp3 + cells. Our results thus demonstrate that endogenous Tregs interact with activated LPS-DCs draining into the LN from the periphery. Prolonged interactions take place near the capsule, and reduce Treg velocity significantly. We infer that such prolonged interactions with immigrant LPS-DCs lead to activation of endogenous Tregs. Treg interactions with DC and Tconv during priming To examine Treg behaviour during an antigen-specific response, we imaged OTII Tconv cells, Ova-pulsed DCs (Ova-DCs) and Tregs at a critical point in T-cell activation, 12 h after the transfer of antigen-specific OTII Tconv cells ( Fig. 4a ). This timing matches the initial formation of naïve CD4 + T-cell clusters around antigen-bearing DCs (phase II of T-cell activation) [16] . As expected, OTII Tconv cells formed clusters around Ova-DCs. We further observed that Tregs form dynamic contacts with both DCs and antigen-specific Tconv cells ( Fig. 4b and Supplementary Video 6 ). Although Tconv cells slowed as they interacted with Ova-DCs, no significant change in Treg velocity was observed compared with steady-state conditions ( Fig. 4c see for example, Fig. 1d ). Treg contact histories illustrate that Tregs spent more time in contact with responding Tconv cells ( Fig. 4d , red bars) than with Ova-DCs (green bars), and were often in contact with both (blue bars). However, in several instances, Tregs transitioned from interacting with both the DC and responding T cell to maintain an interaction with the responding Tconv cell alone ( Fig. 4e and Supplementary Video 8 ). Therefore, during T-cell priming, Tregs engage dynamic clusters of DCs and Tconv cells making frequent, brief contacts but without significant slowing. 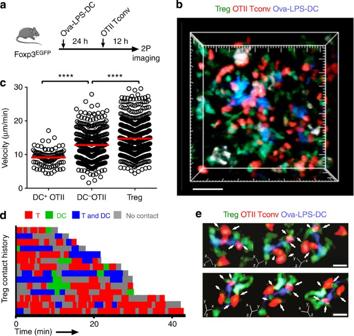Figure 4: Dynamics of Tregs during antigen-specific Tconv priming. (a) Experimental design to examine endogenous Treg behaviour during an immune response. Ova-pulsed DCs were adoptively transferred into Foxp3EGFPmice 24 h prior to transfer of CMTMR-labelled OTII Tconv cells; imaging was performed 12 h after OTII T-cell transfer. (b) Tconv-DC clusters. Still image showing DCs (blue), OTII Tconv cells (red) and Tregs (green). Scale bar, 50 μm, seeSupplementary Video 8. (c) Tconv and Treg velocities. Mean track velocities of OTII T cells were separated into those that interacted with a DC (DC+OTII,n=99) and those that did not (DC−OTII,n=426). Treg velocities,n=811. Data are pooled from three experiments. (d) Contact history map for 14 representative Tregs. Each horizontal bar represents time when a single Treg was alone (grey), in contact with a Tconv (red), in contact with a DC (blue) or in contact with DC:Tconv pairs (green). (e) Close-up images of Treg–Tconv-cell contacts (white arrows) in the vicinity of a DC. The panel shows three-way rotations at two time points, 67 s apart. Scale bar, 10 μm. Figure 4: Dynamics of Tregs during antigen-specific Tconv priming. ( a ) Experimental design to examine endogenous Treg behaviour during an immune response. Ova-pulsed DCs were adoptively transferred into Foxp3 EGFP mice 24 h prior to transfer of CMTMR-labelled OTII Tconv cells; imaging was performed 12 h after OTII T-cell transfer. ( b ) Tconv-DC clusters. Still image showing DCs (blue), OTII Tconv cells (red) and Tregs (green). Scale bar, 50 μm, see Supplementary Video 8 . ( c ) Tconv and Treg velocities. Mean track velocities of OTII T cells were separated into those that interacted with a DC (DC + OTII, n =99) and those that did not (DC − OTII, n =426). Treg velocities, n =811. Data are pooled from three experiments. ( d ) Contact history map for 14 representative Tregs. Each horizontal bar represents time when a single Treg was alone (grey), in contact with a Tconv (red), in contact with a DC (blue) or in contact with DC:Tconv pairs (green). ( e ) Close-up images of Treg–Tconv-cell contacts (white arrows) in the vicinity of a DC. The panel shows three-way rotations at two time points, 67 s apart. Scale bar, 10 μm. Full size image Blocking CTLA4 enhances clustering and limits Treg contacts CTLA4 expressed on Tregs is indispensable for maintenance of immune homoeostasis, and treatment with a blocking antibody leads to T-cell-mediated autoimmune disease [5] , [6] , [7] , [8] . Based on this, we examined the effect of blocking CTLA4 on the dynamics of Tregs during an antigen-specific T-cell response. Using the T-cell priming protocol of Fig. 4 , we injected antigen-primed Foxp3 EGFP mice with αCTLA4 or isotype control (ITC) antibody 30 min after transfer of OTII Tconvs and 4 h before imaging ( Fig. 5a ). OTII Tconv-cell dynamics were visibly altered following αCTLA4 treatment. Stable clusters of OTII T cells formed around Ova-DCs, and Tregs were excluded from these clusters ( Fig. 5b ), thereby reducing Treg interactions with DCs. αCTLA4 treatment enhanced Tconv cluster stability and prevented Tregs from making extensive DC contact ( Supplementary Video 9 ), as indicated by tracks of Tregs and OTII Tconv cells (green and red, respectively, Fig. 5c ) and contact history maps ( Fig. 5d ). In αCTLA4-treated animals, the percentage of OTII Tconv cells that remained in contact with an Ova-DC for over 20 min (stable contact) was significantly higher ( Fig. 5e ). Indeed, OTII Tconv-cell contacts with DCs were significantly longer on average in the presence of αCTLA4 ( P <0.01), whereas Treg interactions with Ova-DCs were not altered ( Fig. 5f ). Collectively, these results indicate that OTII Tconv-cell clustering around Ova-DCs is enhanced by blocking CTLA4. 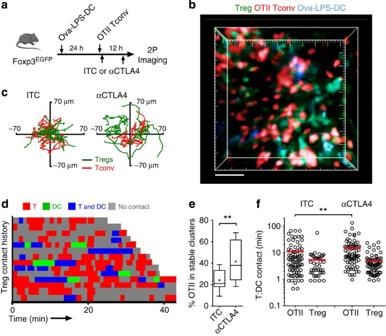Figure 5: Tregs engage antigen-specific clusters of DCs and Tconv cells in a CTLA4-dependent manner. (a) Experimental design to image the role of CTLA4-B7 in Treg interactions. Ova-pulsed DCs from ECFP mice were adoptively transferred into Foxp3EGFPmice 24 h prior to CMTMR-labelled OTII Tconv cells; imaging was performed 12 h after OTII Tconv-cell transfer. Animals received 150 μg of either ITC or αCTLA4, 30 min after adoptive transfer and 4 h prior to imaging. (b) Still image showing DCs (blue), OTII Tconv cells (red) and Tregs (green) in a node from αCTLA4-treated mouse. Scale bar, 50 μm, seeSupplementary Video 9. (c) Superimposed tracks of OTII T cells (red) and Tregs (green), with their origins normalized to the centre of a DC. Cells were tracked for 10:14 (min:s).n=21 for ITC and 34 for αCTLA4. (d) Treg contact history map. Each horizontal bar represents a single Treg, with contacts colour coded as inFig. 4d. Note the shorter red and blue bars as compared withFig. 4d, indicating that Tregs spend less time interacting with Tconv cells and DCs in the presence of αCTLA4. (e) The percentage of OTII T cells in stable contact with a DC was increased by αCTLA4 treatment, compared with control (n=21 and 14, respectively). Imaging period minimum: 20 min. (f) Tconv and Treg contact durations with antigen-bearing DCs. OTII Tconv:DC contact durations are increased in the presence of αCTLA4 (n=78) relative to ITC control (n=80). Treg:DC contact durations were shortened in the presence of αCTLA4 (n=42) relative to ITC (n=83). Figure 5: Tregs engage antigen-specific clusters of DCs and Tconv cells in a CTLA4-dependent manner. ( a ) Experimental design to image the role of CTLA4-B7 in Treg interactions. Ova-pulsed DCs from ECFP mice were adoptively transferred into Foxp3 EGFP mice 24 h prior to CMTMR-labelled OTII Tconv cells; imaging was performed 12 h after OTII Tconv-cell transfer. Animals received 150 μg of either ITC or αCTLA4, 30 min after adoptive transfer and 4 h prior to imaging. ( b ) Still image showing DCs (blue), OTII Tconv cells (red) and Tregs (green) in a node from αCTLA4-treated mouse. Scale bar, 50 μm, see Supplementary Video 9 . ( c ) Superimposed tracks of OTII T cells (red) and Tregs (green), with their origins normalized to the centre of a DC. Cells were tracked for 10:14 (min:s). n =21 for ITC and 34 for αCTLA4. ( d ) Treg contact history map. Each horizontal bar represents a single Treg, with contacts colour coded as in Fig. 4d . Note the shorter red and blue bars as compared with Fig. 4d , indicating that Tregs spend less time interacting with Tconv cells and DCs in the presence of αCTLA4. ( e ) The percentage of OTII T cells in stable contact with a DC was increased by αCTLA4 treatment, compared with control ( n =21 and 14, respectively). Imaging period minimum: 20 min. ( f ) Tconv and Treg contact durations with antigen-bearing DCs. OTII Tconv:DC contact durations are increased in the presence of αCTLA4 ( n =78) relative to ITC control ( n =80). Treg:DC contact durations were shortened in the presence of αCTLA4 ( n =42) relative to ITC ( n =83). Full size image CTLA4-B7 interactions contribute to Treg function CTLA4 is known to negatively regulate T-cell responses through interactions with co-stimulatory B7 molecules, B7.1 (CD80) and B7.2 (CD86) on APCs [31] . In vitro and in vivo studies have shown that Tregs can capture B7 ligands from DCs through a process of trans-endocytosis that requires CTLA4 on Tregs [32] . To determine whether αCTLA4 treatment alters the expression of co-stimulatory ligands on DCs, we transferred LPS-DCs into recipients that were treated with control (ITC) or αCTLA4 antibodies. By flow cytometric analysis, CD80 and CD86 levels were unaffected by αCTLA4 treatment ( Supplementary Fig. 3 ). Although the expression of CD80 and CD86 has been studied most extensively in APCs, we confirm previous observations [33] , [34] , [35] that Tconv cells also express CD86 and upregulate CD80 and CD86 in vivo within 12–24 h of priming ( Supplementary Fig. 4a–d ). Furthermore, after stimulation with anti-CD3/CD28 beads in vitro , CD80 and CD86 were upregulated in Tconv cells that had divided at least once, and elevated levels were retained through several divisions ( Supplementary Fig. 4e ). CTLA4 expression was also increased on Tconv cells that had undergone at least one division, and as expected for activated T cells CD69 expression was significantly increased in proliferating cells ( Supplementary Fig. 5 ). Upregulation of the CTLA4 ligands CD80 and CD86 in Tconv cells suggested that suppressive CTLA4-B7 interactions may not be exclusive to Treg:DC partners, but may contribute to Treg:Tconv interactions. Using αCTLA4-blocking antibody and the same dosing protocol as in Fig. 5a , we first confirmed a previous study [36] that OTII Tconv cells from the draining LNs proliferated more in αCTLA4-treated animals than in ITCs ( Fig. 6a,b ). To complement our results using αCTLA antibody we then used a genetic approach to address whether Tregs mediate CD80/86-dependent Tconv interactions and suppression. We compared proliferation and Treg suppression of WT and CD80/86-double knockout Tconv cells in an APC-free in vitro system (to exclude the effect of Tregs on DCs) using anti-CD3- and anti-CD28-coated beads. WT and CD80/86 knockout Tconv cells proliferated comparably in response to αCD3/CD28 beads ( Fig. 6c ). At a 1:1 ratio, WT Tregs inhibited proliferation of WT Tconvs by 48±1.1% (mean±s.e.m. ); however, Treg suppression was significantly reduced in CD80/86 knockout Tconv cells (38±1.7%, P =0.001, Fig. 6d ). Thus, the lack of CD80/CD86 makes Tconv cells less susceptible to suppression by Tregs. 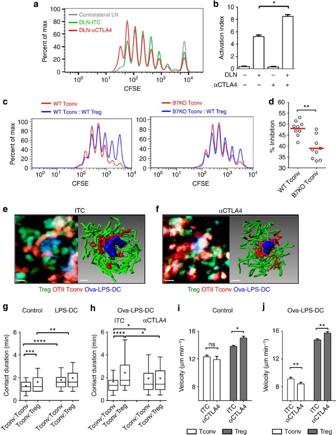Figure 6: CTLA4 is critical for Tconv–Treg interactions during priming. (a) CFSE dilution in OTII Tconv cells 72 h following transfer into WT mice primed with Ova-LPS pulsed DCs. Green and red lines for draining lymph node (DLN) of ITC- and αCTLA4-treated mice, respectively; grey line for contralateral LN with αCTLA4. (b)In vivoproliferation of OTII Tconv determined by CFSE dilution; data from four to five mice with αCTLA4 or ITC control treatment. (c)In vitroproliferation of Tconv (WT, left, and B7-KO, right) after stimulation with anti-CD3/28 Dynabeads with (blue) and without (red) WT Treg co-culture (1:1). (d) Inhibition of WT and B7-KO Tconv-cell proliferation by WT Tregs; red bars indicate mean values, data pooled from two independent experiments. (e) Left: Ova-pulsed DCs (blue) interacting with OTII Tconvs (red) and Tregs (green) in a Foxp3EGFPmouse. Right: tracks of Tconvs and Tregs that touched a DC at least once during imaging (20:55 (min:s)); tracks normalized to DC position; scale bar, 10 μm. (f) Left: Ova-pulsed DCs (blue), OTII Tconvs (red) and Tregs (green) in Foxp3EGFPmouse treated with αCTLA4. Right: tracks of Tconvs and Tregs that interacted with a DC (blue) at least once during imaging (20:33 (min:s)). Scale bar, 10 μm. (g) Contact durations of OTII Tconvs in the absence and presence of LPS-DCs. Basal: Tconv:Tconv,n=135; Tconv:Treg,n=234. LPS-DCs present: Tconv:Tconv,n=108; Tconv:Treg,n=145. (h) Contact durations of OTII Tconvs in the presence of Ova-pulsed DCs after treatment with 150 μg isotype control (ITC) or αCTLA4 antibodies. ITC treated: Tconv:Tconv,n=101; Tconv:Treg,n=108. αCTLA4 treated: Tconv:Tconv,n=87; Tconv:Treg,n=152. (i) Velocities of OTII Tconvs and Tregs under basal conditions after treatment with ITC or αCTLA4 antibodies. Tconv tracks:n=268 (ITC) and 238 (αCTLA4); Treg tracks:n=296 (ITC) and 213 (αCTLA4). (j) Velocities of OTII Tconvs and Tregs in Ova-LPS-DC immunized mice after treatment with ITC or αCTLA4 antibodies. Tconv tracks:n=99 (ITC) and 114 (αCTLA4). Treg tracks:n=811 (ITC) and 305 (αCTLA4). NS, not significant. Figure 6: CTLA4 is critical for Tconv–Treg interactions during priming. ( a ) CFSE dilution in OTII Tconv cells 72 h following transfer into WT mice primed with Ova-LPS pulsed DCs. Green and red lines for draining lymph node (DLN) of ITC- and αCTLA4-treated mice, respectively; grey line for contralateral LN with αCTLA4. ( b ) In vivo proliferation of OTII Tconv determined by CFSE dilution; data from four to five mice with αCTLA4 or ITC control treatment. ( c ) In vitro proliferation of Tconv (WT, left, and B7-KO, right) after stimulation with anti-CD3/28 Dynabeads with (blue) and without (red) WT Treg co-culture (1:1). ( d ) Inhibition of WT and B7-KO Tconv-cell proliferation by WT Tregs; red bars indicate mean values, data pooled from two independent experiments. ( e ) Left: Ova-pulsed DCs (blue) interacting with OTII Tconvs (red) and Tregs (green) in a Foxp3 EGFP mouse. Right: tracks of Tconvs and Tregs that touched a DC at least once during imaging (20:55 (min:s)); tracks normalized to DC position; scale bar, 10 μm. ( f ) Left: Ova-pulsed DCs (blue), OTII Tconvs (red) and Tregs (green) in Foxp3 EGFP mouse treated with αCTLA4. Right: tracks of Tconvs and Tregs that interacted with a DC (blue) at least once during imaging (20:33 (min:s)). Scale bar, 10 μm. ( g ) Contact durations of OTII Tconvs in the absence and presence of LPS-DCs. Basal: Tconv:Tconv, n =135; Tconv:Treg, n =234. LPS-DCs present: Tconv:Tconv, n =108; Tconv:Treg, n =145. ( h ) Contact durations of OTII Tconvs in the presence of Ova-pulsed DCs after treatment with 150 μg isotype control (ITC) or αCTLA4 antibodies. ITC treated: Tconv:Tconv, n =101; Tconv:Treg, n =108. αCTLA4 treated: Tconv:Tconv, n =87; Tconv:Treg, n =152. ( i ) Velocities of OTII Tconvs and Tregs under basal conditions after treatment with ITC or αCTLA4 antibodies. Tconv tracks: n =268 (ITC) and 238 (αCTLA4); Treg tracks: n =296 (ITC) and 213 (αCTLA4). ( j ) Velocities of OTII Tconvs and Tregs in Ova-LPS-DC immunized mice after treatment with ITC or αCTLA4 antibodies. Tconv tracks: n =99 (ITC) and 114 (αCTLA4). Treg tracks: n =811 (ITC) and 305 (αCTLA4). NS, not significant. Full size image CTLA4 stabilizes Treg interactions with Tconv cells Collectively, the above results point towards an important functional role of Treg CTLA4 interactions with CD80/86 on Tconvs. To examine the choreography of these interactions, we compared Treg:Tconv interactions under control conditions (ITC) and following αCTLA4 treatment. In ITC-treated mice, it was clear that Tregs interacted extensively with Tconvs, while also simultaneously interacting with DCs during antigen priming ( Fig. 6e ). In contrast, during αCTLA4 treatment Tregs did not interact with Tconv in DC clusters ( Fig. 6f ). To quantitatively analyze the role of CTLA4 in stabilizing T-cell–T-cell interactions, we measured contact durations under steady-state, inflammatory and priming conditions. Steady-state Tconv:Treg cell contacts, although brief, were significantly longer than Tconv:Tconv-cell contacts ( Fig. 6g ). Treg interaction times with Tconvs were prolonged in the presence of LPS-DCs, implying that inflammatory conditions may increase Tconv:Treg adhesion ( Fig. 6g ). During antigen activation of OTII Tconv cells, Tconv:Treg interaction times were substantially increased, and notably αCTLA4 treatment during priming reduced Tconv:Treg contact durations to steady-state values ( Fig. 6h ). These results indicate that the prolonged interactions between Tconv and Tregs during inflammation and priming are CTLA4 dependent. In light of the high constitutive expression of CTLA4 by Tregs and induced expression of CTLA4 by Tconvs, as well as apparently conflicting evidence as to whether CTLA4 over-rides or has no effect on the TCR-induced stop-signal [37] , [38] , we also analyzed the effects of αCTLA4 treatment on OTII Tconv and Treg velocities under both steady-state and priming conditions. In the absence of cognate antigen, αCTLA4 treatment increased Treg velocity modestly without significantly altering Tconv-cell velocity ( Fig. 6i ). Under priming conditions, DC-interacting OTII Tconv velocities were reduced by αCTLA4 treatment, while at the same time Treg velocities were increased relative to ITC treatment ( Fig. 6j ). These results are consistent with the well-known observation that velocities are reduced by cellular interactions as cells cluster during priming [14] , [16] . Previous in vitro and in vivo studies have described both contact-dependent and cytokine-mediated mechanisms of suppression by Tregs [11] , [39] , [40] . In this study, we employed 2P imaging to directly visualize and characterize the behaviour of endogenous Tregs and their interactions with DCs and Tconvs. Two non-overlapping populations of Tregs were observed in LN: one in the T-cell zone and one in the follicle. The follicular population was characterized by its position near the periphery of the LN, colocalization with B cells and lack of exchange with Tregs in the T-zone as defined by colocalization with Tconv cells. fTregs have been previously described as being retained in the B-cell follicle by expression of CXCR5 + and high local concentrations of CXCL13 (ref. 24 ), and have been shown to regulate germinal centre formation [25] . Here we focus on T-zone Tregs that limit Tconv-cell priming. Several imaging studies used in vitro -expanded T cells to infer the effects of Tregs on Tconv cells in LN, but without a full consensus on mechanisms of immunoregulation [17] , [18] , [21] . Tadokoro et al . [18] concluded that Tregs inhibit CD4 + helper T-cell interactions with DCs; Angiari et al . [21] found that Treg inhibition of T-cell:DC contacts and cluster formation was restricted to the late phases of activation; whereas Mempel et al . [17] observed that the addition of Tregs did not affect the long duration interactions between CD8 + cytotoxic T lymphocytes and antigen-presenting B-cell targets. Tang et al . [19] imaged adoptively transferred antigen-specific CD4 + CD25 + Tregs during immune response to islet antigen and concluded that DC–Treg interactions limit helper T-cell activation. Recently, Pace et al . [22] indirectly demonstrated that Tregs suppress low-avidity CD8 + responses to foreign antigens, showing that Treg depletion did not alter the long lasting APC–T-cell interactions induced by high-affinity antigen, whereas short duration interactions induced by low affinity antigen were prolonged. While reporting the role of Mst 1 kinase in Tregs, Tomiyama et al . [20] suggested an alternative mechanism that antigen-specific Tregs downregulate co-stimulatory molecules on DCs but are unlikely to inhibit naïve T-cell priming by physically competing for DCs. However, in that study [20] 2P imaging was performed on sliced LN instead of intact or in vivo LN, raising caveats regarding damage to tissue architecture. Distinct from previous studies, our results provide evidence for direct physical interaction among endogenous Tregs with Tconv and APCs during an ongoing immune regulation in LN and further highlight the role of CTLA4 in coordinating these interactions. 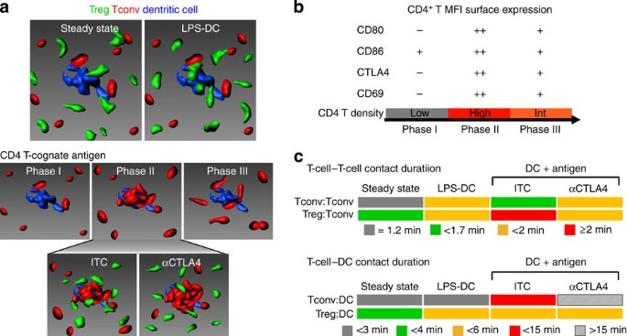Figure 7: Summary of Treg, Tconv and DC dynamics. (a) Cellular choreography illustrating cell dynamics and the role of CTLA using cell shapes rendered from 2P images (Tregs, green; Tconv, red; DCs, blue). Panels represent steady-state conditions (top left); inflammation (LPS DC; top right); T-cell priming in three phases (middle); Tregs interacting with clusters during phase II under normal priming conditions (labelled ITC for isotype control, bottom left) and in the presence of CTLA4-blocking antibody (labelled αCTLA4, bottom right). (b) Chart of relative surface expression by Tconv cells during T-cell priming. CD4 density refers to the local concentration of antigen-specific T cells near antigen-presenting DCs during phase II. (c) Colour-coded diagram of measured contact durations among Tregs and Tconvs (top panel), and among T cells and DCs (bottom panel). Each change in contact duration (different colours) represents a significant difference of at leastP<0.05. Figure 7 depicts a summary of cellular choreography, surface markers and cell interactions measured by contact durations under basal conditions, during inflammation and during T-cell priming. Figure 7: Summary of Treg, Tconv and DC dynamics. ( a ) Cellular choreography illustrating cell dynamics and the role of CTLA using cell shapes rendered from 2P images (Tregs, green; Tconv, red; DCs, blue). Panels represent steady-state conditions (top left); inflammation (LPS DC; top right); T-cell priming in three phases (middle); Tregs interacting with clusters during phase II under normal priming conditions (labelled ITC for isotype control, bottom left) and in the presence of CTLA4-blocking antibody (labelled αCTLA4, bottom right). ( b ) Chart of relative surface expression by Tconv cells during T-cell priming. CD4 density refers to the local concentration of antigen-specific T cells near antigen-presenting DCs during phase II. ( c ) Colour-coded diagram of measured contact durations among Tregs and Tconvs (top panel), and among T cells and DCs (bottom panel). Each change in contact duration (different colours) represents a significant difference of at least P <0.05. Full size image Under basal conditions in the absence of antigen ( Fig. 7a top left), Tconv cells move rapidly and in a random-walk search for cognate antigen, sampling DCs with brief interactions [41] . In the present study, we show that Tregs in the T-cell zone migrate even faster than Tconv cells and engage both resident DCs and Tconv cells in frequent, brief contacts. Tregs have elongated processes, and contacts with Tconv are characterized by close apposition of membranes. Although Tregs constitute only 5–10% of the total number of T cells in the LN, our data indicate that individual Tconvs and resident DCs interact directly with Tregs with high frequency, and are in contact with at least one Treg 36 and 47% of the time under basal conditions. During inflammation ( Fig. 7a top right), activated DCs from the periphery enter the LN via afferent lymphatics and encounter Tregs near the LN capsule. Activated DCs not pulsed with exogenous antigen upregulate CD80 and CD86, and present self-antigens in the context of MHCII refs 29 , 42 . We demonstrate that activated LPS-DCs form prolonged contacts with Tregs and that the presence of LPS-DCs causes a significant increase in the proportion of Tregs that are activated. The interactions of Tregs with LPS-activated DCs are reminiscent of prolonged CD4 T-cell interactions with dermally derived antigen-presenting DCs during priming [16] . When antigen is present on migratory DCs ( Fig. 7a bottom), the cellular dynamics undergo marked changes that can be divided into three phases as previously described [16] . We show the dynamic behaviour and physical interaction of Tregs with Tconvs and DCs during phase II (sustained contact). During this phase, Tregs frequently interact with clusters of APC:Tconv but remain highly motile, suggesting that Tregs transiently scan these clusters. Our results complement a recent study reporting interaction behaviour of antigen-specific Tregs with CTLs and APCs in a tumour model [43] . That study and our results suggest that APCs displaying peptide–MHC complexes and co-stimulatory molecules provide a platform for Tconv and Treg interaction. Mechanistically, Tregs have been proposed to regulate immune responses by decreasing CD80 and CD86 on APCs in a CTLA4 dependent manner, thus rendering APCs less potent for further activation of Tconv cells [32] , [44] , [45] , [46] . However, in our experiments, in vivo treatment with αCTLA4 did not alter expression of the co-stimulatory ligands, CD80 and CD86 in adoptively transferred and LN-recovered DCs. Several in vitro APC-free assays have shown that Tregs are capable of direct inhibition of Tconv-cell activation in a contact-dependent and antigen-independent manner [12] , [47] . We confirm this, and now provide direct evidence for CTLA4-dependent physical interactions between Treg:Tconv cells during immune activation in vivo . Coinciding with phase II of antigen-specific Tconv priming, when cognate Tconv cells interact stably with DCs and high-density Tconv:DC clusters form (8–16 h), we show that Tconv cells increase their expression of CD80 and CD86 on activation ( Fig. 7b ), becoming potential targets for CTLA4-mediated interaction with Tregs. In the presence of blocking αCTLA4 antibody, Tregs appeared oblivious to both DCs and Tconvs, resulting in larger and more stable Tconv:DC clusters and contributing to enhanced T-cell proliferation in vivo . Contact-dependent suppression mediated by B7 molecules on activated T cells was previously proposed by Paust and Cantor [39] . CD86 is expressed by naïve CD4 + T cells, and we demonstrate that both CD80 and CD86 are expressed by activated CD4 + T cells. Using an in vitro , APC-free, genetic approach we show that lack of CD80 and CD86 expression on Tconvs renders them less susceptible to suppression by Tregs. Notably, Treg suppression is not completely abrogated, because multiple mechanisms for Treg suppression of Tconv-cell priming may operate simultaneously [11] , [48] , [49] . Here we show that CTLA4 on Tregs limits Tconv clustering around antigen-bearing DCs. We demonstrate that Tregs physically engage Tconv cells that have upregulated CD80 and CD86. Indeed, we found that αCTLA4 treatment disrupts both Treg–Tconv and Treg–DC cell interactions at this early time point of T-cell activation ( Fig. 7c ). Moreover, T-cell–T-cell synapses have been reported to play a critical role in CD8 T-cell differentiation through active exchange of cytokines during transient T–T synapse formation [50] . In line with a recent report on the role of CTLA4 in stabilizing Treg synapses in vitro [51] , our study delineates an important functional role of Tregs to limit priming through CTLA4 interactions with upregulated B7 ligands on Tconv cells in vivo . Finally, it has been suggested that CTLA4 may play a role in the inhibition of TCR-induced T-cell stopping [37] , [52] , but this is controversial [38] . In our study, treatment with αCTLA4 increased steady-state Treg motility while having no effect on Tconv motility. During antigen-specific immune activation, treatment with αCTLA4 again enhanced Treg motility, but antigen-specific Tconv exhibited a significant decrease in velocity while forming stable clusters with DCs. Considering the role of CTLA4 in stabilizing Treg immune-synapses [51] , local exclusion of Tregs when CTLA4 is blocked could contribute to enhanced Tconv-cell clustering adjacent to DCs. Mice, cell labelling and reagents Mice were housed in a clean, pathogen-free facility. Animal care and protocols were reviewed and approved by Institutional Animal Care and Use Committee of the University of California, Irvine and the animal ethics committee of Ghent University (ethical committee number 2013-015), in accordance with European guidelines (directive 2010/63/EU; Belgian Royal Decree of 6 April 2010). Male mice from the C57Bl/6 background were used at 8–12 weeks of age in donor/recipient experiments. Foxp3 EGFP mice expressing enhanced GFP along with Foxp3 were obtained from Jackson Laboratories (Stock Number 006772). The CD11c–EYFP mouse strain expressing enhanced YFP on the CD11c promoter [26] was a kind gift from M. Nussenzweig (The Rockefeller University, New York, NY, USA). Foxp3 EGFP male mice were crossed with CD11c EYFP female mice to generate F1 heterozygote females. Other mouse strains included β-actin–cyan fluorescent protein (β-actin–CFP; Stock Number 004218), TCR transgenic ova-IA b -specific OTII mice (Stock Number 004194), CD80 −/− CD86 −/− mice (Stock Number 003610) and WT C57Bl/6 mice (Stock Number 000664) were purchased from Jackson Laboratories. Cell labelling was performed by suspending 4–6 million cells in 4 ml of RPMI-1640 at 37 °C, quenching and washing twice with RPMI-1640 containing 10% FBS (Gibco). Tconv cells were labelled with 10 μM 5-(and-6)-(((4-chloromethyl)benzoyl)amino)tetramethylrhodamine (CMTMR) for 30 min; for proliferation assays OTII Tconv cells were labelled with 1.6 μM carboxyfluorescein succinimidyl ester (CFSE) for 7 min; in some analyzed videos (not shown) DCs were labelled blue with 40 μM CMF 2 HC for 40 min (Molecular Probes, CellTrace series). The following antibodies were purchased from BioLegend and were used at 0.2 μg ml −1 for flow-cytometry and 100 μg per animal for in vivo blocking: anti-mouse CTLA4 (clone 9H10, Syrian hamster IgG), ITC (hamster IgG), anti-mouse CD4 (clone GK1.5), APC-conjugated anti-mouse Vα2 (clone B20.1), anti-mouse CD69, anti-mouse CD62L, anti-mouse CD80 (clone 16-10A1) and anti-mouse CD86 (clone GL1). All adoptive transfers were performed under anaesthesia and mild restraint, via tail-vein injection (T cells) or by subcutaneous injection (DCs) near a draining LN. DC culture and Tconv-proliferation assays Bone marrow-derived DCs for 2P imagining were generated as described [53] . Briefly, marrow was extracted from the femur of 6–10-weeks-old mice and cultured in non-tissue culture-treated polystyrene dishes for 9–10 days (Corning) using RPMI-1640 (Lonza) supplemented with 1% L-glutamine, 10% foetal calf serum (Hyclone Inc.), 100 U ml −1 penicillin, 100 μg ml −1 streptomycin, 2-βME and GM-CSF, IL-4 and TNFα, as previously described [53] . For in vivo proliferation assays, IL-4 and TNFα were excluded to enhance antigen uptake during Ova-pulsing. For activated DCs and antigen-specific T–DC interaction imaging studies, DCs were treated with LPS (100 ng ml −1 ) alone or with LPS+Ova (100 μg ml −1 ) for 12–24 h prior to harvest and injection. CD4 + CD25 − T cells (Tconv) were isolated from spleen and LNs of 6–10-week-old mice using negative selection (Miltenyi Biotec and StemCell Technologies). For APC-free in vitro proliferation, CFSE-labelled WT Tconv cells were co-cultured with anti-CD3/CD28-coated dynabeads (Life Technologies) at 1:1 ratio according to the manufacturer’s protocol. Tregs were added to Tconv at 1:1 ratio for suppression assays. CFSE dilution in live cells (Fixable Viability Dye eFluor 780 negative gating; eBioscience) was analyzed using BD LSRII flow cytometer. For measuring the effects of αCTLA4 on in vivo proliferation, 2 × 10 6 Ova-DCs were injected subcutaneously into the footpad of WT mice; after 18 h 3 × 10 6 CFSE-labelled OTII Tconv cells were injected intravenously; popliteal LNs were collected on day 3 of Tconv-cell transfer; LN from the contralateral hind limb served as immunization control. CFSE dilution in single cells was analyzed by gating on Vα2 + CFSE + population. Activation indices (AI) were calculated using equation (1), as described [54] , where M values correspond to the number of cell divisions assessed by CFSE dilution. 2P imaging All images were acquired with excitation wavelengths between 890 and 910 nM. Two imaging systems were used. The primary system used is a custom-built 2P system based on an Olympus BX5 upright microscope, with excitation generated by a tunable Chameleon femtosecond laser (Coherent). Dichroic filters (495 and 560 nm) were arranged in series to separate blue, green and red signals, and images were collected as previously described [55] at UC-Irvine. EGFP and EYFP signals are separated using a 520 nm dichroic filter. Additional data were collected on a Zeiss inverted 710 2-photon system in the Inflammation Research Center (IRC), VIB-U Gent with a Zeiss SP 485 nm, LP 490 nm, LP 555 nm, BP 565–610 nm filter combination arranged in series with blue, green and red photomultiplier tubes. Both microscopes were fitted with either a × 20 (numerical aperture (NA)=0.95), × 25 (NA=1.05) or × 60 (NA=1.1) water-immersion objectives, and equipped with three photomultiplier tubes, peristaltic heated perfusion systems (Warner Instruments) and thermocouple-based temperature sensors placed next to the tissue. All imaging was carried out on LNs maintained at 37°±0.5 °C and superfused with RPMI-1640 and medical grade carbogen gas (95% O 2 and 5% CO 2 ). Size and velocity comparisons of endogenous Foxp3–EGFP T cells from each microscope were analyzed separately and found to be nearly identical with no significant variation. Data analysis All image analysis was performed using Imaris software (Bitplane) version 6.5–7.2. Cells were tracked manually and contact durations were measured with three-dimensional rotation to verify contacts. Stable contact formation was defined as any OTII T cell that remained in contact with one DC for a minimum of 20 min. Unless otherwise noted, displayed images in all figures are maximal intensity projections through the z -axis (‘top view’) of x – y – z stacks. Flow-cytometry was performed on either a BD LSRII (UC-Irvine and VIB-UGent) or BD LSR-Fortessa (VIB-UGent) and analyzed using FlowJo. Figures were generated using Graphpad Prism and OriginPro8. Statistical analysis was performed using Mann–Whitney test (unpaired sample, nonparametric); P values are marked in figures: * P <0.05; ** P <0.01; *** P <0.001 and **** P <0.0001. How to cite this article: Matheu, M. P. et al . Imaging regulatory T cell dynamics and CTLA4-mediated suppression of T cell priming. Nat. Commun. 6:6219 doi: 10.1038/ncomms7219 (2015).